Dynamic encoding of face information in the human fusiform gyrus Humans’ ability to rapidly and accurately detect, identify and classify faces under variable conditions derives from a network of brain regions highly tuned to face information. The fusiform face area (FFA) is thought to be a computational hub for face processing; however, temporal dynamics of face information processing in FFA remains unclear. Here we use multivariate pattern classification to decode the temporal dynamics of expression-invariant face information processing using electrodes placed directly on FFA in humans. Early FFA activity (50–75 ms) contained information regarding whether participants were viewing a face. Activity between 200 and 500 ms contained expression-invariant information about which of 70 faces participants were viewing along with the individual differences in facial features and their configurations. Long-lasting (500+ms) broadband gamma frequency activity predicted task performance. These results elucidate the dynamic computational role FFA plays in multiple face processing stages and indicate what information is used in performing these visual analyses. Face perception relies on a distributed network of interconnected and interactive regions that are strongly tuned to face information [1] . One of the most face selective regions in the brain is located in fusiform gyrus (the fusiform face area, FFA). Damage to FFA results in profound impairments in face recognition [2] , and the FFA is thought to be a processing hub for face perception [3] . Recent studies have demonstrated that the FFA activity contains information about individual faces invariant across facial expression [3] and gaze/viewpoint [4] , and have started to describe some of the organizing principles of individual-level face representations [5] , [6] , [7] . However, due to the use of low temporal resolution analyses or imaging modalities, little is known regarding the relative timing of when FFA becomes sensitive to different aspects of face-related information. Specifically, face processing is thought to occur through a set of partially distinct stages [8] , and it remains unclear in which of these stages FFA participates and, more generally, when they occur in the brain. Evidence from FFA in humans and the putative analogue to FFA in non-human primates has demonstrated that FFA shows strong selectivity for faces versus non-face objects [9] , [10] , [11] , [12] , [13] , [14] . There is disagreement about when exactly the FFA, and the human brain in general, first responds selectively to faces [15] , [16] , [17] . In particular, it is unknown when FFA becomes face selective relative to areas in lateral occipital cortex [15] , [16] , [18] , relative to single neurons in the cortex of non-human primates [12] , [13] , [14] , [19] and relative to rapid behavioural face detection [20] . A recent study using intracranial electrocorticography (ECoG) showed that fusiform becomes sensitive to the category of a visual object around 100 ms after stimulus onset [21] . However, the brain network highly tuned to face information [1] may allow faces to be processed more rapidly than other categories of objects. Therefore, it remains unclear how early FFA becomes face selective and whether it contributes to face detection. Regarding face individuation, ensembles of single neurons responsive to individual faces have been identified in face-sensitive cortical regions of the non-human primate brain [13] , [14] , [22] , [23] . Studies with humans also show that FFA encodes information about individual faces [3] , [6] . However, little is known regarding the temporal dynamics of individual face processing in FFA, particularly relative to other processing stages. Furthermore, it remains unknown whether FFA is sensitive to the key facial features used for face recognition, particularly the eyes, mouth and configural face information. Single neurons of middle face patch in the non-human primate (a putative homolog of FFA) show sensitivity to external facial features (face aspect ratio, direction, hair length and so on) and properties of the eyes [22] . A recent ECoG study showed that FFA is sensitive to global and external features of the face and head (face area, hair area and so on) [6] . Behavioral studies have shown that the eyes are the most important facial feature used for face recognition, followed by the mouth [24] and that configural and holistic processing of faces is correlated with face recognition ability [25] . It remains unknown whether FFA is sensitive to individual differences in these featural and configural properties critical to face recognition, particularly when changeable aspects of the face (for example, expression) are taken into account. Finally, how FFA contributes to task-related stages of face processing is undetermined. Specifically, previous studies have described a late, long-lasting (lasting many hundreds of milliseconds) face specific broadband gamma frequency (40+Hz) activity [6] , [26] , [27] . Broadband gamma activity is closely related to the underlying population firing rates [28] , [29] , both of which are face selective for many hundreds of milliseconds after seeing a face [14] , [26] , [27] , extending well beyond the timeframe of face individuation seen in non-human primates [14] . It is unknown what role this long-lasting activity plays in face processing. Here we examine whether this long-lasting gamma band activity reflects the maintenance of face information in support of perceptual decision-making and working memory processes [30] , [31] . We used intracranial ECoG in humans and multivariate machine learning methods to document the temporal dynamics of face information processing in the FFA from the moment a face is first viewed through response-related processing. Multivariate pattern classification was used to decode the contents and timecourse of information processing in FFA to elucidate the dynamics and computational role of this area in face perception. Electrophysiological activity (specifically the timecourse of the single-trial voltage potentials and broadband gamma frequency power) from the epileptically unaffected FFA was assessed, while each of four patients (P1-4) participated in two face processing experiments (see Fig. 1 for electrode locations; all face-sensitive electrodes appear to be in mid-fusiform, lateral to the mid-fusiform sulcus, see Weiner et al. [2014] for a detailed description regarding the face-sensitive regions of the fusiform). Experiment 1 was adopted to examine the temporal dynamics of face sensitivity and specificity in FFA (for example, face detection), and experiment 2 was employed to examine the temporal dynamics of face individuation and categorization invariant with respect to facial expression. The results of these experiments demonstrate that, within 75 ms of presentation, FFA activity encodes the presence of a face (face detection), between 200 and 450 ms FFA activity encodes which face it is (face individuation), and late (500+ ms) broadband gamma FFA activity encodes task-related information about faces. These results demonstrate the dynamic contribution of FFA to multiple, temporally distinct face processing stages. 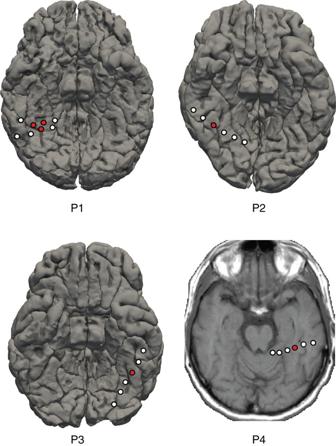Figure 1: Locations of electrodes used in the study and their neighbouring electrodes on subjects’ native pial surface reconstruction. Electrodes in red denote the ones used in the experiment and electrodes in white denote the other contacts on the same electrode strip. A high resolution MRI was not available for pial surface reconstruction of P4, and thus the electrode is visualized on a low resolution T1 MRI slice. MNI coordinates of electrodes are as follows: P1—(35, −59, −22), (33, −53, −22), (42, −56, −26); P2—(40, −57, −23); P3—(−33, −44, −31); P4—(−38, −36, −30). All electrodes are over the fusiform gyrus. Figure 1: Locations of electrodes used in the study and their neighbouring electrodes on subjects’ native pial surface reconstruction. Electrodes in red denote the ones used in the experiment and electrodes in white denote the other contacts on the same electrode strip. A high resolution MRI was not available for pial surface reconstruction of P4, and thus the electrode is visualized on a low resolution T1 MRI slice. MNI coordinates of electrodes are as follows: P1—(35, −59, −22), (33, −53, −22), (42, −56, −26); P2—(40, −57, −23); P3—(−33, −44, −31); P4—(−38, −36, −30). All electrodes are over the fusiform gyrus. Full size image Timecourse and magnitude of face sensitivity in FFA To assess the face sensitivity and specificity of FFA (experiment 1), we used a k-nearest neighbours algorithm to decode the neural activity while participants viewed six different categories of visual images: faces, human bodies, houses, hammers, shoes and phase-scrambled faces (30 images per category, each repeated once, presented in random order; faces, bodies and shoes were balanced for gender; see Fig. 2a for examples). Participants pressed a button if an image was repeated in consecutive trials (20% of trials, repeated images were excluded from analysis). Each individual participated in two sessions of experiment 1; one session from P4 was not used due to evidence of an ictal event during the recording (a total of seven sessions across four participants). We classified single-trial voltage potentials between 100 and 250 ms after stimulus presentation into one of the six categories described above and examined the decoding accuracy using the signal recorded from face-sensitive electrodes (see Methods for details on electrode selection and Fig. 1 for locations). This time range was selected for the initial analysis because it includes most of the previously described face-sensitive electrophysiological responses [9] , [15] , [26] (also see Fig. 2a,b ). We were able to identify the category of a stimulus presented on a given trial with 54–93% accuracy across the seven sessions if the stimulus was a face (six-way classification, chance=16.7%). Neural activity for non-face images was misclassified as a face in 0–8% across the sessions (P1=93/0%, 82/1%; P2=88/8%, 54/8%; P3=73/6%, 77/1%; P4=67/8%; true-positive rate/false-positive rate; chance=16.7/16.7%; P <10 −5 in each of the eight sessions). Little consistency in classification accuracy was seen across sessions and participants for the five other object categories ( Supplementary Table 1 ). In addition, in all participants electrodes 1-2 cm away from the electrodes of interest showed little face-sensitive (peak sensitivity index [ d ′] <1, Fig. 1 and Supplementary Fig. 1 ), suggesting that face sensitivity was constrained within 1–2 cm. The high sensitivity and specificity for face classification reported here demonstrates that human FFA regions are strongly face selective [14] , [19] . 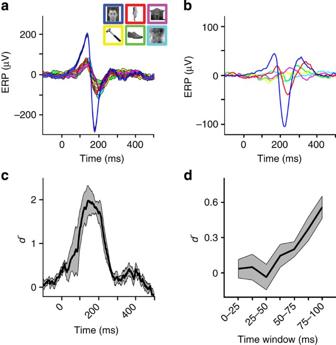Figure 2: Dynamics of face selectivity in human FFA. (a) Example of stimuli from each condition and event related potential (ERP) waveforms from session 1 of P1. Across trial means are plotted and standard errors are shaded in light colours. (b) Average ERP waveforms across the four participants. In each participant a positive going face-sensitive peak between 100 and 140 ms and a negative going face-sensitive peak between 160 and 200 ms could be identified. The timing of these peaks is consistent with previous ERP studies of face processing9,15,26. (c) Face classification accuracy over time as measured byd′ (n=4, meand′ plotted against the beginning of the 100 ms sliding window), which takes into account both the true- and false-positive rate. Classification is based on single-trial voltage potentials. SeeSupplementary Fig. 1for individual subjectd′ timecourses for these electrodes and neighbouring electrodes. Standard deviations are shaded grey. (d) Face classification accuracy in the first 100 ms after stimulus onset with 25 ms windows. Classification is based on single-trial voltage potentials.d′ scores in panelscandddiffer due to the different window sizes used for the respective analyses. s.d. values are shaded grey. Figure 2: Dynamics of face selectivity in human FFA. ( a ) Example of stimuli from each condition and event related potential (ERP) waveforms from session 1 of P1. Across trial means are plotted and standard errors are shaded in light colours. ( b ) Average ERP waveforms across the four participants. In each participant a positive going face-sensitive peak between 100 and 140 ms and a negative going face-sensitive peak between 160 and 200 ms could be identified. The timing of these peaks is consistent with previous ERP studies of face processing [9] , [15] , [26] . ( c ) Face classification accuracy over time as measured by d ′ ( n =4, mean d ′ plotted against the beginning of the 100 ms sliding window), which takes into account both the true- and false-positive rate. Classification is based on single-trial voltage potentials. See Supplementary Fig. 1 for individual subject d ′ timecourses for these electrodes and neighbouring electrodes. Standard deviations are shaded grey. ( d ) Face classification accuracy in the first 100 ms after stimulus onset with 25 ms windows. Classification is based on single-trial voltage potentials. d ′ scores in panels c and d differ due to the different window sizes used for the respective analyses. s.d. values are shaded grey. Full size image Figure 2c shows the temporal dynamics of single-trial face classification averaged across participants in FFA using the sensitivity index ( d ′), which takes into account both the true- and false-positive rate for face detection. Face sensitivity was seen in FFA between ~50 and 350 ms after stimulus onset. To determine the onset of face selective activity in FFA, we examined the d ′ for face classification from 0 to 100 ms in 25 ms moving windows shifted by 12.5 ms. All windows between 50 and 100 ms showed significant face sensitivity ( Fig. 2d , 50–75 ms: mean d ′=0.200, t (3)=3.13, P =0.0260; 62.5–87.5 ms: mean d ′=0.368, t (3)=3.72, P =0.0169; 75–100 ms: mean d ′=0.551, t (3)=5.91, P =0.0048), earlier time windows did not reach statistical significance. None of the other five categories, including phase scrambled faces, showed significant classification in these time windows. This suggests that this rapid face processing was not driven by spatial frequency information [17] as phase scrambled faces contain the same spatial frequency content as intact faces. The 50–75 ms time window is earlier than human fusiform becomes sensitive to other visual object categories [21] . However, this time window is consistent with the reports of the earliest face sensitivity in single cortical neurons in non-human primates [12] , [13] , [14] , [19] and rapid behavioural face detection [20] , suggesting that FFA is involved in face detection. Timecourse of individual-level face processing in FFA In each of two sessions recorded on separate days, P1-P4 were shown 70 different faces, each repeated five times with different facial expressions each time (happy, sad, angry, fearful and neutral expressions) for a total of 350 unique images. The participants’ task was to report the gender of each face they saw (50% male, 50% female faces). We used a nearest neighbour classification algorithm to determine how accurately we could predict which face (given two drawn from the set of faces) a participant was viewing at a particular moment in session 1 based on a model trained on the timecourse of the single-trial voltage potentials from session 2. Session 2 was used as the training set and session 1 as the test set for this analysis to test classification on previously unseen faces. In each of the four participants in experiment 2, above chance intra-session classification of the neural response to individual faces was observed ( Fig. 3a , P <0.05 using a permutation test, corrected for multiple time comparisons). Classification accuracy peaked in P1 at 65% and was significant in the 210–390 ms time window, in P2 at 59% and was significant in the 280–460 ms time window, in P3 at 63% and was significant in the 270–490 ms time window, and in P4 at 60% and was significant in the 350–540 ms time window (chance=50%; 57% corresponds to P =0.05 corrected for multiple comparisons). In addition, we examined whether individual-level face classification was invariant over expression by training the classifier on four of the five expressions and testing the other, then repeating this with different expressions in the training and test set until each expression (leave-one-expression-out cross-validation). In each participant, above chance across-expression classification of the neural response to individual faces was observed ( Fig. 3b , P <0.05 using a permutation test, corrected for multiple time comparisons). This across-expression classification had a similar timecourse as the across-session classification in Fig. 3a , suggesting that the coding for individual faces in FFA is not driven by low-level differences between images and is at least partially invariant over expression. Indeed, classification of expression failed to reach statistical significance at any point between 0 and 500 ms ( Supplementary Fig. 5 ). In addition, classification accuracy across face genders was similar to classification within face gender ( Supplementary Fig. 6 ), suggesting that classification of individual faces in FFA was not driven by task demands. Also, training with the data from session 1 and classifying the data from session 2 changed the peak classification accuracy by <0.5%, the peak time by <15 ms and the significant time window by <25 ms. Furthermore, individual faces could not be classified above chance in the adjacent or nearby electrodes ( Supplementary Fig. 7 ). These results suggest that the 200–500 ms time window is critical for expression-invariant face individuation in FFA. 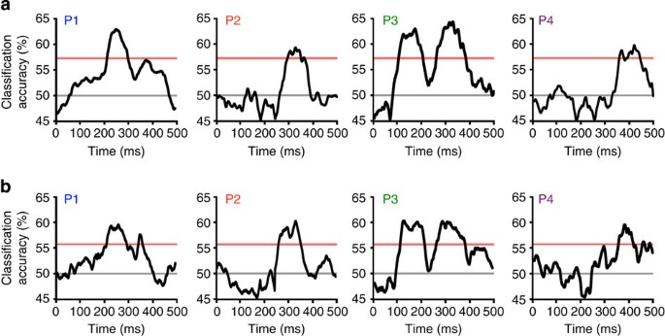Figure 3: Face individuation in human FFA. (a) Time course of individual level face classification accuracy based on single-trial voltage potentials in each participant. This shows, given two faces, how accurately we could predict which one the participant was viewing based on the neural data, plotted against the beginning of the 100 ms sliding window. Red line at 57% indicatesP=0.05, corrected for multiple time comparisons based on the permutation test, grey line indicates chance accuracy (50%). (b) Across-expression, individual level face classification accuracy. This shows, given two faces with a particular expression, how accurately we could predict which one the participant was viewing based on the neural data from the other four expressions used in the study. Red line at 55.5% indicatesP=0.05, corrected for multiple time comparisons based on the permutation test, grey line indicates chance accuracy (50%). Figure 3: Face individuation in human FFA. ( a ) Time course of individual level face classification accuracy based on single-trial voltage potentials in each participant. This shows, given two faces, how accurately we could predict which one the participant was viewing based on the neural data, plotted against the beginning of the 100 ms sliding window. Red line at 57% indicates P =0.05, corrected for multiple time comparisons based on the permutation test, grey line indicates chance accuracy (50%). ( b ) Across-expression, individual level face classification accuracy. This shows, given two faces with a particular expression, how accurately we could predict which one the participant was viewing based on the neural data from the other four expressions used in the study. Red line at 55.5% indicates P =0.05, corrected for multiple time comparisons based on the permutation test, grey line indicates chance accuracy (50%). Full size image Facial information used in service of face individuation To investigate what specific face information FFA encodes in the service of face individuation, we mapped anatomical landmarks on each of the faces presented in experiment 2 and projected each face into an 18-dimensional ‘feature space’ that applied to all faces (for example, eye area, nose length, mouth width, skin tone and so on; see Fig. 4 for a full list of the features used) [32] . The multivariate canonical correlation between these facial feature dimensions and the voltage potentials between 200 and 500 ms post-stimulus onset was then calculated to evaluate the shared relationship between these variable sets. The full canonical model between the neural activity and the face feature space was significant in P1, P3 and P4 and approached significance in P2 (P1: χ 2 (171)=211.33, Wilks’ λ =0.021, P =0.019; P2: χ 2 (152)=181.21, Wilks’ λ =0.045, P =0.053; P3: χ 2 (171)=230.93, Wilks’ λ <0.001, P =0.001; P4: χ 2 (152)=194.06, Wilks’ λ =0.03, P =0.012) demonstrating that FFA activity is sensitive to individual differences in these facial feature dimensions. Only the full model was significant as none of the other hierarchical statistical tests reached significance. 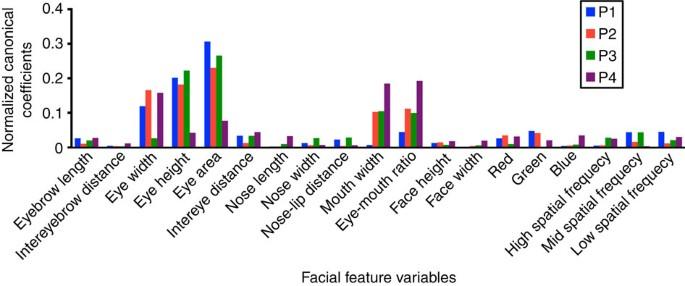Figure 4: Facial feature sensitivity of FFA electrodes. Multivariate canonical correlation coefficients between the single-trial voltage potentials and facial features for the individual faces. Canonical coefficients have a similar interpretation as beta coefficients in multiple regression. Coefficients were normalized by first taking the absolute value and then dividing by the sum of all coefficients across the 18 facial feature variables. Figure 4 presents the normalized function weights for the full canonical model demonstrating that the most relevant facial variables were related to the eyes, the mouth, and the ratio between eye and mouth dimensions. There are also notable differences across participants, with P1 showing strong sensitivity to eye information and almost no sensitivity to mouths and P4 showing strong sensitivity to mouth information and less to eyes. It is unclear whether these differences are due to different electrode locations (see Fig. 1 ), random variation (as we do not have the power with only four participants to statistically quantify these individual differences) or different face processing strategies among participants. More generally, we did not track eye movements and therefore cannot relate our results to particular face processing strategies or preclude FFA sensitivity to other internal or external facial features [6] , [22] . Rather our results show that, under free viewing conditions, FFA is tuned to natural variations in eye and mouth feature dimensions and configural information relating the eyes to the mouth in service of face individuation. Figure 4: Facial feature sensitivity of FFA electrodes. Multivariate canonical correlation coefficients between the single-trial voltage potentials and facial features for the individual faces. Canonical coefficients have a similar interpretation as beta coefficients in multiple regression. Coefficients were normalized by first taking the absolute value and then dividing by the sum of all coefficients across the 18 facial feature variables. Full size image Broadband gamma activity predicts task performance Finally, we examined the role of the slowly decaying broadband gamma power (40–90 Hz) activity that has been shown to be face sensitive [6] , [26] , [27] . The results from experiment 1 confirm that this gamma activity shows strong selectivity for faces and also showed that it lasts for the entire trial ( Fig. 5a and Supplementary Fig. 8 ). Experiment 1 was a working memory task, and one possible role for face-specific activity that persists for the entire trial is task-related maintenance of face information that is manipulated by frontal and/or parietal regions involved in working memory and decision making [30] , [31] , [33] . In support of this hypothesis, in repeated trials face activity decayed more rapidly than in first presentations, potentially due to the release of task demands once detection was accomplished. However, the relative paucity of repeated face trials and decreased face activity due to repetition suppression make interpreting these results difficult. Thus, to test the hypothesis that broadband gamma frequency activity was related to maintaining the face representation in support of task-related processing, we examined the relationship between long-lasting gamma activity and behavioural reaction time in experiment 2. In support of a role in task-related processing, the decay time of the gamma activity from 500 to 1,000 ms after stimulus presentation predicted reaction time in experiment 2. Specifically, longer lasting gamma activity was significantly correlated with slower response times ( P <0.05) in the gender identification task for each participant ( Figs 5b and 6a ). The amplitude of this gamma band activity 100–300 ms before the response significantly predicted reaction time for each participant, and this activity returned to baseline only once the participants had responded and task demands had waned ( Figs 5c and 6b ). While this gamma frequency power significantly predicted reaction time, we were unable to decode the gender decision of the participant from this activity. In summary, greater than baseline, face-specific broadband gamma power was seen until the point of behavioural response, and a larger gamma peak and more rapid decay predicted more rapid decisions of face gender, but this gamma activity did not predict behavioural responses (that is, ‘male’ or ‘female’). 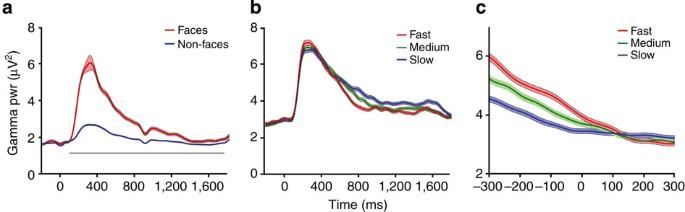Figure 5: Long-lasting task-related broadband gamma activity. (a) Mean and s.e. of gamma band (40–90 Hz) power for face and non-face trials across all participants in experiment 1 (n=4). Grey bar indicatesP<0.05 for face versus non-face objects based on the Wilcoxon rank–sum test. SeeSupplementary Fig. 8for face and non-face gamma band power for each individual participant. (b) Mean and s.e. of gamma band power split into thirds by reaction time for gender discrimination in experiment 2 (n=4; mean reaction time=P1: 788 ms; s.d.=269 ms; P2: 870 ms; s.d.=221 ms; P3: 1,065 ms; s.d.=299 ms; P4: 872 ms; s.d.=216 ms). Significant correlation was seen in each individual participant between 500–1,000 ms gamma band power and reaction time (Fig. 6a). (c) Same as for (b) but with trials aligned to the behavioural response (time 0=response onset) for the four participants in experiment 2. A significant correlation between pre-response gamma band power (−300 to −100 ms) and reaction time was seen in each individual participant (Fig. 6b). Figure 5: Long-lasting task-related broadband gamma activity. ( a ) Mean and s.e. of gamma band (40–90 Hz) power for face and non-face trials across all participants in experiment 1 ( n =4). Grey bar indicates P <0.05 for face versus non-face objects based on the Wilcoxon rank–sum test. See Supplementary Fig. 8 for face and non-face gamma band power for each individual participant. ( b ) Mean and s.e. of gamma band power split into thirds by reaction time for gender discrimination in experiment 2 ( n =4; mean reaction time=P1: 788 ms; s.d.=269 ms; P2: 870 ms; s.d.=221 ms; P3: 1,065 ms; s.d.=299 ms; P4: 872 ms; s.d.=216 ms). Significant correlation was seen in each individual participant between 500–1,000 ms gamma band power and reaction time ( Fig. 6a ). ( c ) Same as for ( b ) but with trials aligned to the behavioural response (time 0=response onset) for the four participants in experiment 2. A significant correlation between pre-response gamma band power (−300 to −100 ms) and reaction time was seen in each individual participant ( Fig. 6b ). 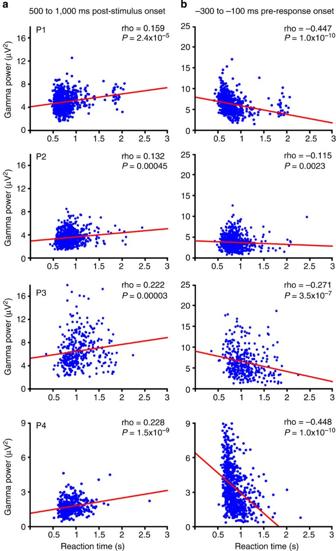Figure 6: Gamma power predicts reaction time in each participant. (a) Scatter plots of mean gamma power over the 500–1,000 ms post stimulus window versus reaction time. (b) Scatter plots of mean gamma power over the −100 to −300 ms pre response window versus reaction time. Red line indicates best fit regression line. Full size image Figure 6: Gamma power predicts reaction time in each participant. ( a ) Scatter plots of mean gamma power over the 500–1,000 ms post stimulus window versus reaction time. ( b ) Scatter plots of mean gamma power over the −100 to −300 ms pre response window versus reaction time. Red line indicates best fit regression line. Full size image Our results establish the timecourse of information processing in human FFA and elucidate the specific computations FFA performs on faces from the moment a face is first viewed through decision-related processing. These results demonstrate that FFA activity first contains face-specific information ~50–75 ms after subjects viewed a face. FFA displays sharp face sensitivity between 100 and 250 ms, with little evidence for selectivity for four other categories of non-face objects or phase scrambled faces. Individual-level face information invariant over facial expression could be decoded for previously unseen faces between 200 and 500 ms. During this same time window, the neural activity from FFA contained information about individual differences in eye and mouth features and the relative size of eyes versus mouths, suggesting that the FFA uses this information to individuate faces. Finally, late, long-lasting (500+ms) gamma frequency band activity (40–90 Hz) predicted participants’ trial-by-trial reaction times in a gender categorization task. Taken together, these results reveal the highly dynamic role that FFA plays in multiple distinct stages of face processing. One caveat of the current work is that the input to all of our analyses was the timecourse of FFA activity recorded from single electrodes in each participant. The significant decoding demonstrated in this analysis suggests that FFA displays at least a degree of temporal encoding of face information [34] . However, the data we report are only weakly sensitive to information that is primarily coded spatially. Specifically, the data are differentially sensitive to neural populations with different proximity or different orientations relative to the electrodes. That said information primarily encoded spatially is far less likely to be detected by our analyses than information encoded temporally. Thus, lack of significant classification (for example, for expression or the gender decision) does not necessarily imply that FFA is not sensitive to this information, but rather it is not coded temporally. FFA is face sensitive in the 50–75 ms time window. This time window is as early (or earlier) as face sensitivity in lateral occipital face-sensitive regions [15] , [18] and is consistent with onset of face sensitivity reported for single cortical neurons in non-human primates [12] , [13] , [14] , [19] . Behaviourally, it has been shown that humans can saccade towards a face within 100–150 ms (ref. 20 ). The decoding of face information in the 50–75 ms time window reported here is consistent with FFA playing a role in this rapid face detection. The early face sensitivity of FFA reported here provides strong evidence that this area is involved in face detection. A recent human ECoG study showed that category selective activity is first observed in temporal cortex around 100 ms after stimulus onset [21] . Our results show that human FFA becomes face sensitive in the 50–75 ms window, suggesting that faces are processed more rapidly in temporal cortex than other object categories. Indeed, studies of single-neuron firing latencies in non-human primates have reported that face sensitivity first arises around the 50–75 ms window [12] , [13] , [14] , [19] . This more rapid processing of face information may be a result of the network of areas highly tuned to face properties [1] . Future studies will be required to determine whether non-face categories with highly tuned perceptual networks (for example, words [35] and bodies [36] ) are also processed more rapidly than other categories of objects. One caveat is that the ECoG study by Liu et al. [21] reported that the 100 ms object category response in temporal cortex shows invariance to viewpoint and scale changes and future studies will be required to determine whether the 50–75 ms FFA face-sensitive response is invariant over these transformations as well. The time window critical for individual level classification occurred between 200 and 500 ms, after face sensitivity observed in experiment 1 had mostly waned. One potential explanation why face individuation occurred during a period where face-specific activity is relatively weak is that individual level face information may be represented by relatively few neurons (sparse coding) [37] . Sparse coding would imply that relatively few face-sensitive neurons were active and that the summed face-related activity in this time period therefore would be weak. However, the neurons that were active encode for individual level face information, which would explain the significant decoding of identity we report here. One point to note is that, while face-specific voltage potentials had waned in this time period, significant face-specific broadband gamma activity was observed in the same time period as individual level face classification, though it too was declining. To the extent that this broadband gamma activity reflects single-neuron firing [28] , [29] , the decrease in this activity potentially also supports a sparse coding hypothesis. One caveat being that further studies are required to determine whether the decrease in broadband gamma is due to less neurons being active in this time period (sparse coding) or a decrease in the firing rate. Neuroimaging studies and lesion studies in patients have implicated parts of anterior temporal cortex strongly connected to the FFA [38] , [39] as important to face individuation [3] , [40] , [41] . Furthermore, a recent study suggested that FFA might act as a hub of face identity processing and act in concert with these anterior temporal face-sensitive regions [3] . The timewindow in which we found individual-level face coding (200–500 ms) is generally consistent with the idea that recurrent top-down and bottom-up interactions are likely to be critical to face individuation. Note that in P3 and perhaps in P1 there are two peaks of individual-level face classification. More data will be required to statistically substantiate these two peaks; however, the dual peaks suggest the possibility of a feedback loop involved in face individuation. Neural activity in FFA during the same time window when significant individual-face decoding was observed (200–500 ms) displayed significant multivariate correlation to variation in the eyes, mouth and eye-mouth ratio. Behavioural studies have shown that the eyes are the most important facial feature used for face recognition, followed by the mouth [24] and that holistic and configural face processing ability is correlated with face recognition [25] . A recent study revealed that electrical stimulation of FFA distorts the perception of facial features [42] . Furthermore, previous studies have demonstrated the importance of the presence of the eyes for face perception in general, and FFA activity in particular [43] . Our results lend strong evidence to the hypothesis that FFA uses individual differences in these facial features in service of face individuation and recognition. We show that FFA shows face-specific gamma frequency power that lasts until task demands wane and that the amplitude of this power predicts participants’ reaction times. Recent studies demonstrate that long-lasting FFA gamma activity is modulated by task-related attention to faces and facial expression [26] , [27] , in support of the hypothesis that this activity is integral to task-performance. While this activity did predict reaction time, it did not predict the gender decision. This suggests that FFA supports task-related processing, potentially by keeping face information on-line, but decision-specific processing occurs elsewhere, likely in frontal and parietal regions using the information from FFA [30] , [31] . Indeed, a recent study challenged the view that frontal areas store working memory and task-relevant information and suggested that these areas instead control and manipulate information that is stored elsewhere [33] . In the case of faces our results suggest that at least some of this information is stored in FFA. In summary, our results provide strong evidence that the FFA is involved in three temporally distinct, but partially overlapping processing stages: face detection, expression-independent individuation using facial features and their configuration, and task-related gender classification. Information about these processing stages was present in the recordings from electrodes within a 1 cm radius in each participant suggesting that the same, or at least very nearby, neural populations are involved in these multiple information processing stages. A key open question is how processing transitions between stages in these local neural populations. One hypothesis is that the dynamics of these processing stages are governed by interactions between multiple regions of the face processing network. Taken together with previous findings, the current results suggest a model in which FFA contributes to the entire face processing sequence through computational analysis of multiple aspects of face information at different temporal intervals. Subjects The experimental protocols were approved by the Institutional Review Board of the University of Pittsburgh. Written informed consent was obtained from all participants. Four human subjects underwent surgical placement of subdural electrode grids and ventral temporal electrode strips as standard of care for surgical epilepsy localization. P1 was male, age 26, and had seizure onset in the hippocampus. P2 was female, age 30, and had seizure onset in the frontal lobe. P3 was female, age 30, and had seizure onset in premotor cortex. P4 was male, age 65, and had seizure onset in the hippocampus. None of the participants showed evidence of epileptic activity on the FG electrode used in this study. The order of the participants (P1–P4) is chronological, based on their recording dates. Stimuli In experiment 1, 30 images of faces (50% male), 30 images of bodies (50% male), 30 images of shoes (50% mens’ shoes), 30 images of hammers, 30 images of houses and 30 images of phase scrambled faces were used. Phase scrambled images were created in Matlab by taking the two-dimensional spatial Fourier spectrum of the image, extracting the phase, adding random phases, recombining the phase and amplitude, and taking the inverse two-dimensional spatial Fourier spectrum. Each image was presented in pseudorandom order and repeated once in each session. Faces in experiment 2 were taken from the Karolinska Directed Emotional Faces stimulus set [44] . Frontal views and five different facial expressions (happy, sad, angry, fearful and neutral) from all 70 faces (50% male) in the database were used for a total of 350 face images, each presented once in random order during a session. Owing to time and clinical considerations, P3 was shown 40 faces (50% male) from the database for a total of 200 faces each presented once in random order during a session. All stimuli were presented on an LCD computer screen placed ~2 m from participants’ heads. Experimental paradigms In experiment 1, each image was presented for 900 ms with 900 ms inter-trial interval during which a fixation cross was presented at the centre of the screen (~10° × 10° of visual angle). At random, 20% of the time an image would be repeated. Participants were instructed to press a button on a button box when an image was repeated (1-back). Only the first presentations of repeated images were used in the analysis. In experiment 2, each face was presented for 1,500 ms with 500 ms inter-trial interval during which a fixation cross was presented at the centre of the screen. Subjects were instructed to report whether the face was male or female via button press on a button box. Each individual participated in two sessions of experiment 2 on different days. Paradigms were programmed in Matlab using Psychtoolbox and custom written code. Data preprocessing Data were collected at 2,000 Hz. They were subsequently bandpass filtered offline from 1 to 115 Hz using a second order Butterworth filter to remove slow and linear drift, the 120 Hz harmonic of the line noise and high frequency noise. Data were also notch filtered from 55 to 65 Hz using a second order Butterworth filter to remove line noise. To reduce potential artefacts in the data, trials with maximum amplitude 5 s.d. values above the mean across the rest of the trials were eliminated. In addition, trials with a change of >25 μV between consecutive sampling points were eliminated. These criteria resulted in the elimination of <6% of trials in each subject. Electrode localization Coregistration of iEEG electrodes used the method of ref. 45 . High resolution CT scans of patients with implanted electrodes are combined with anatomical MRI scans before neurosurgery and electrode implantation. The Hermes method accounts for shifts in electrode location due to the deformation of the cortex by utilizing reconstructions of the cortical surface with FreeSurfer software and co-registering these reconstructions with a high-resolution post-operative CT scan. It should be noted that electrodes on the ventral surface typically suffer minimal shift as compared with those located near the craniotomy. A cortical surface reconstruction was not possible in P4 due to the lack of a high-resolution MRI. Instead the high-resolution post-operative CT scan was transformed into MNI space using a low resolution T1 MRI and the electrode locations manually determined. Electrode selection Electrodes were chosen based on anatomical and functional considerations. Electrodes of interest were restricted to those that were located on the fusiform gyrus. In addition, electrodes were selected such that their peak six-way face classification d ′ score (see below for how this was calculated) exceeded 1.5 and the ERP for faces was larger than the ERP for the other object categories. To avoid concerns about circularity with regards to electrode selection, only the data from the training set (odd trials, see below) for the classification results reported were used for electrode selection. Thus, all statistical values and classification accuracies reported for 6-way face classification are derived from data independent of those used for electrode selection and classifier training. This procedure yielded one electrode per participant, except for P1 where it yielded three nearby electrodes (see Supplementary Fig. 1 ). In the case of P1, we averaged the signal from the three face-sensitive electrodes (all three electrodes are shown in Fig. 1 ). For P2 the third electrode displayed a peak d ′>1.5; however, in examining the ERP it was evident that face classification accuracy in the third electrode on the strip was due to lesser face activity relative to the other conditions (see Supplementary Fig. 4 ). Face classification on the fourth electrode for P2 was also above threshold and the activity in this electrode followed the pattern from other subjects (for example, greater face activity relative to other conditions), thus we chose this electrode. It should be noted that even if the anatomical restriction was lifted and all electrodes were used, no additional electrodes would have been chosen in any participant. In addition to the four participants included in the study, six other individuals participated in the experimental paradigm during the study period. None of these individuals had any electrodes that met the selection criteria and thus were not included in the analysis. In two of these individuals, there were no electrodes on ventral temporal cortex. The electrode locations from the four excluded participants with ventral temporal cortex electrodes are shown in Supplementary Fig. 2 . In one of these individuals, data quality was poor (excessive noise) for unknown reasons (EP2, none of the electrodes showed any visual response and were anterior to FFA). In three of these individuals, data quality was reasonable and there were electrodes on ventral temporal cortex, yet none met the selection criteria (see Supplementary Fig. 3 ). In one of the non-included participants one electrode exceeded the d ′ threshold (see Supplementary Fig. 3 ), but this was due to lesser face activity relative to the other conditions (see Supplementary Fig. 4 ). Considering the ventral electrode strips are placed without functional or anatomical/visual guidance, a yield of 4/7 individuals with ventral strip electrodes having electrodes placed over highly face selective regions is a substantial yield. Experiment 1 classification analysis and statistics For classification, single-trial potentials were first split into odd trials used as the training set and even trials used as the test set. The Euclidean distance between the time windowed data from each of the test and each of the training trials was then calculated. The single-trial potentials from the test trial were assigned to the stimulus condition with k-nearest neighbours classifier. Alternatively, using the correlation (instead of Euclidean distance) between the test and training sets, the results yielded were not substantively different. The selection of k was determined by finding the greatest d ′ for k-nearest neighbour classification based on random sub-sampling validation with 50 repeats using only the training set. True-positive and false alarm rates were calculated across all of the test trials. The d ′ was calculated as Z (true-positive rate)— Z (false alarm rate), where Z is the inverse of the Gaussian cumulative distribution function. As training and test data were separated (rather than cross validation) and not reversed (for example, the training and test sets were not switched), there is no statistical dependence between the training and test sets and classification accuracy follows the binomial distribution. The null hypothesis for statistical testing was that the true-positive rate was equal to the false-positive rate under the binomial distribution (this justifies the use of a one tailed t -test). Experiment 2 classification analysis and statistics To determine whether information regarding individual faces was present in the timecourse of the single-trial potentials, we used across sessions binary nearest neighbours classification (for example, k =1). Specifically, the neural responses for the five presentations (each with a different facial expression) of two faces in the second session were used as the training set. The test set was the average signal across the five presentations of one of those faces in the first session. The Euclidean distance between the single-trial potentials from the test face and each training face in a 100 ms window was calculated. The test neural activity was classified as belonging to the face that corresponded to the neural activity in the training set that was closest to the neural activity from the test trial. This procedure was then repeated for all possible pairs of faces and all time windows slid with 5 ms steps between 0 and 500 ms after the presentation of the face. It should be noted that single-trial classification was also examined, and, while classification accuracy was lower, it was still as statistically significant in each participant as when using the average activity across expressions for the 70 face identities (statistical significance was higher due to the use of 350 individual trials instead of 70 averaged trials, which increased statistical power, 40 faces and 200 trials in P3). In addition, cross-expression classification was also calculated using the same classifier and time windows as above. In this case the neural response for the eight presentations of four of the expressions (four expressions × two sessions) of two faces were used as the training set. The test set was the average signal across the two presentations of the remaining expressions for one of those faces in the first session. This procedure was repeated for each pair of faces and with each expression left out as the test set (for example, leave-one-expression-out cross-validation). Note that, using cross-validation, instead of holdout validation as in the cross-session classification, and analyzing the five expressions separately, lowered the statistical threshold for this analysis. Permutation testing was used for statistical testing of classification accuracy in experiment 2. Specifically, the labels of the faces in each session were randomly permuted. The same procedure as above was performed on these permuted trials. The maximum classification accuracy across the 0–500 ms time window was then extracted. Using the maximum classification accuracy across the time window implies a global null hypothesis over the entire window, which corrects for multiple time comparisons [46] . The labels were randomly permuted again and this procedure was repeated 500 times. Using this procedure, P =0.05, corrected for multiple comparisons, corresponded to a classification accuracy of ~57% (±0.2% across the four individuals). Classification of the five facial expressions ( Supplementary Fig. 5 ) was done using k -nearest neighbours as in experiment 1. Classification accuracy when the two training faces were the same gender or when they were different gender was also compared in Supplementary Fig. 6 . This was done because participants’ task was gender classification and we wanted to address the potential concern that neural classification for individual faces could have been driven by task demands. Facial feature analysis Facial features were determined based on anatomical landmarks found by IntraFace [32] . This toolbox marks 49 points on the face along the eyebrows, down the bridge of the nose, along the base of the nose, and outlining the eyes and mouth. On the basis of these landmarks we calculated the first 12 facial feature dimensions listed in Fig. 3b . Red, green and blue intensities were calculated by taking the average intensity for these colours in two 20 × 20 pixel squares, one on each cheek, the bottom of which was defined to align with the bottom of the nose and the middle to horizontally align with the middle of the eye. High, middle and low spatial frequencies were determined by calculating the mean power at different levels of a Laplacian pyramid [47] . The image was iteratively low-pass filtered and subtracted from the original image to generate a six-level Laplacian pyramid (from level 0 to level 5), similar to two-dimensional wavelet decomposition. The level with smaller index contained higher frequency components. By adding up in pairs, for example, level 0&1, level 2&3, level 4&5, we get three images that corresponding to the high, mid and low frequency components of the original image (note that if we add all six levels together we will get the original image). We then performed a two-dimensional Fast Fourier Transform for these three images to calculate the mean power for each of them. The values for these 18 feature dimensions were averaged across the five facial expressions for each of the 70 faces (40 for P3). Finally, the values for each variable were normalized by subtracting the mean and dividing by the s.d. across the 70 faces so that none would unduly influence the canonical correlation analysis. Canonical correlation analysis Canonical correlation analysis (CCA) finds the maximally correlated linear combinations of two multidimensional variables [48] , in this case variable one was the 18 facial feature dimensions and variable two was the single-trial potentials between 200 and 500 ms after stimulus onset. In brief, the first canonical coefficients (a 1 m and b 1 n ) of the face and neural variables (x 1 , x 2 , …, x m and y 1 , y 2 , …, y n ), respectively, are found by maximizing the correlation between the canonical variables (W 1 and V 1 ) defined by: This procedure is then repeated for W 2 and V 2 to W p and V p where P =min( m ,i) and all Ws are uncorrelated to one another and all Vs are uncorrelated to find subsequent canonical coefficients and functions. Significance of Wilks’ λ (the multivariate generalization of the inverse of R 2 ) was based on the chi-squared statistic. In the presence of noise, CCA is prone to overfit the data unless the number of samples substantially exceeds the dimensionality of the data. To reduce the dimensionality of the neural data, we performed a principal components analysis (PCA) on the faces × timepoints data (70 faces × 300 time points) and used the first N eigenvalues as the neural dimensions in the CCA. The number of eigenvalues ( N ) was chosen such that they accounted for 90% of the variance in the neural data. This yielded nine eigenvalues for P1, eight for P2, nine for P3 and eight for P4. Gamma band analysis and statistics Time-frequency power spectra were calculated using a Fourier transform with a Hanning window taper calculated with a 200 ms sliding window and 2 Hz frequency step for each trial. The peak frequency in the gamma range for all trials in experiment 1 collapsed across conditions and subjects was found to be 65 Hz, and a window of +/−25 Hz around this peak was used as the frequency window of interest. Trials in experiment 2 were ranked by reaction time (RT) and split into fastest, middle and slowest thirds according to RT. In addition, Spearman’s rho between RT and gamma power across trials was calculated. Spearman’s rho was used to minimize the potential for outliers skewing the correlation, though it should be noted that Pearson’s correlation and Spearman’s rho did not substantially differ in any participants and both were significant in all runs and participants. How to cite this article: Ghuman, A. S. et al. Dynamic encoding of face information in human fusiform. Nat. Commun. 5:5672 doi: 10.1038/ncomms6672 (2014).